RETRACTED ARTICLE: TRIB2 confers resistance to anti-cancer therapy by activating the serine/threonine protein kinase AKT Intrinsic and acquired resistance to chemotherapy is the fundamental reason for treatment failure for many cancer patients. The identification of molecular mechanisms involved in drug resistance or sensitization is imperative. Here we report that tribbles homologue 2 (TRIB2) ablates forkhead box O activation and disrupts the p53/MDM2 regulatory axis, conferring resistance to various chemotherapeutics. TRIB2 suppression is exerted via direct interaction with AKT a key signalling protein in cell proliferation, survival and metabolism pathways. Ectopic or intrinsic high expression of TRIB2 induces drug resistance by promoting phospho-AKT (at Ser473) via its COP1 domain. TRIB2 expression is significantly increased in tumour tissues from patients correlating with an increased phosphorylation of AKT, FOXO3a, MDM2 and an impaired therapeutic response. This culminates in an extremely poor clinical outcome. Our study reveals a novel regulatory mechanism underlying drug resistance and suggests that TRIB2 functions as a regulatory component of the PI3K network, activating AKT in cancer cells. The emergence of drug-resistant tumour cells is a major obstacle for both conventional chemotherapeutics as well as novel targeted therapeutics [1] . As FOXO proteins play a key role in the action of several anticancer drugs, proteins that are capable of suppressing FOXO activity are strong candidates to confer drug resistance [2] , [3] , [4] , [5] , [6] , [7] . Our previous large scale genetic screen identified the kinase-like protein Tribbles 2 ( TRIB2 ) as a FOXO suppressor protein [8] , while TRIB2 has also been implicated in the development and progression of melanoma and leukaemia [8] , [9] , [10] , [11] . In our study presented here, we describe a new regulatory mechanism underlying drug resistance in different cancer entities and suggests that TRIB2 functions as a critical regulatory component of the PI3K signalling network, activating AKT in cancer cells. In addition, our data support the use of TRIB2 as a biomarker for both prognosis and personalized cancer therapy, as well as identifying this protein as a molecular target for combination cancer treatment. 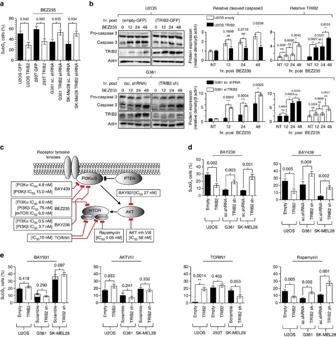Figure 1: Overexpression of TRIB2 confersin vitroresistance to PI3K inhibitors. (a) Matched isogenic TRIB2 cell line FACS analysis following exposure to BEZ235 (n=6), sc.shRNA indicates scramble shRNA while TRIB2 shRNA indicates stable shRNA knockdown for TRIB2 in each cell lines.Pvalues are indicated for each comparison by two-way analysis of variance (ANOVA) and data represent the mean±s.d. (b) (left) Higher pro-caspase3 and reduced cleavage of caspase3 in TRIB2 overexpressing cells after treatment with BEZ235, (50 μg total protein loaded per lane and separated by 10% SDS–PAGE). (right) Densitometry for cleaved caspase3 and TRIB2 under each condition. Data normalized to actin and analysed in ImageJ. Data indicates relative mean intensity±s.e.m and analysed by two-way ANOVA. (c) Schematic showing the target specificity for each compound, the inhibitory concentration 50% (IC50) and commercial name. (d) FACS analysis of TRIB2 isogenic cell lines 72 h post exposure to various pre-clinical PI3K inhibitors (n=6). (e) Isogenic TRIB2 cell line FACS analysis 72 h post-AKT, mTOR1/2 or mTOR1 inhibition (n=6).Pvalues are indicated for each comparison by two-way analysis of variance (ANOVA) and data represent the mean±s.d. TRIB2-conferred resistance to anti-cancer therapeutics To test our hypothesis that the TRIB2 protein confers resistance to anti-cancer drugs, we first generated and then examined the sensitivity of several stable, isogenic TRIB2 in vitro models ( Supplementary Table 1 ; Supplementary Fig. 1 ) after treatment with the dual PI3K/mTOR kinase inhibitor BEZ235. High-TRIB2 expression significantly increased cell resistance to BEZ235 treatment characterized by a significantly lower sub-G 1 cell population and a reduction of caspase-3 cleavage ( Fig. 1a,b ). To characterize the profile of kinases that were affected by TRIB2 status, we tested a range of inhibitors that display distinct kinase selectivity (summarized in Fig. 1c ). TRIB2 protein expression significantly influenced isogenic cell line sensitivity to BAY236 (BAY 80-6946) and BAY1082439 treatment ( Fig. 1d ). This response was independent of the cell cycle ( Supplementary Fig. 2a–c ), indicating that TRIB2 reduces cell death induced by PI3K inhibitors and thus is capable of conferring resistance to these drugs. Strikingly, isogenic cell line sensitivity to inhibition of the central effector protein AKT (ref. 12 ) and to the mTORC1/2 inhibitor TORIN1 was independent of TRIB2 status ( Fig. 1e ). We investigated this further and exposed our isogenic cell lines to rapamycin, a specific mTORC1 inhibitor. Noticeably, TRIB2 status correlated with resistance to this compound ( Fig. 1f ). Taken together our data raises the intriguing possibility that TRIB2 acts upstream of these proteins affecting AKT and mTORC2. Figure 1: Overexpression of TRIB2 confers in vitro resistance to PI3K inhibitors. ( a ) Matched isogenic TRIB2 cell line FACS analysis following exposure to BEZ235 ( n =6), sc.shRNA indicates scramble shRNA while TRIB2 shRNA indicates stable shRNA knockdown for TRIB2 in each cell lines. P values are indicated for each comparison by two-way analysis of variance (ANOVA) and data represent the mean±s.d. ( b ) (left) Higher pro-caspase3 and reduced cleavage of caspase3 in TRIB2 overexpressing cells after treatment with BEZ235, (50 μg total protein loaded per lane and separated by 10% SDS–PAGE). (right) Densitometry for cleaved caspase3 and TRIB2 under each condition. Data normalized to actin and analysed in ImageJ. Data indicates relative mean intensity±s.e.m and analysed by two-way ANOVA. ( c ) Schematic showing the target specificity for each compound, the inhibitory concentration 50% (IC 50 ) and commercial name. ( d ) FACS analysis of TRIB2 isogenic cell lines 72 h post exposure to various pre-clinical PI3K inhibitors ( n =6). ( e ) Isogenic TRIB2 cell line FACS analysis 72 h post-AKT, mTOR1/2 or mTOR1 inhibition ( n =6). P values are indicated for each comparison by two-way analysis of variance (ANOVA) and data represent the mean±s.d. Full size image TRIB2 protein level correlates with AKT activation To investigate this further, we performed western blot analyses before and after clinically representative drug treatment with each compound using our isogenic cell lines. We note a prominent TRIB2-dependent disparity in the levels of pSer473-AKT1 and total AKT using our in vitro models. In melanoma and osteosarcoma cells with high-TRIB2 protein expression, we identified significantly higher levels of total AKT and pSer473-AKT and the opposite was observed in cancer cells with TRIB2 depletion ( Fig. 2a ). Consistent with our previous data, this was not observed for pThr308-AKT1, where there were readily detectable levels of this AKT isoform independent of TRIB2 status in each in vitro model. These data support the intriguing possibility that TRIB2 might promote the further activation of AKT via Ser473 phosphorylation in a PI3K and mTORC1 independent manner. In this way, drugs targeting these proteins within the PI3K pathway are not effective in tumours where TRIB2 expression is up-regulated. To investigate this possibility, we analysed signalling components within the PI3K/AKT network and found that TRIB2 over expression increased the activation of pSer473-AKT before and in the presence of PI3K and mTOR inhibitors ( Fig. 2b ). Importantly, while TRIB2 protein over expression significantly increased pSer473-AKT1 levels, isogenic cell line exposure to our inhibitor compounds reduced the level of pSer473-AKT, indicating that the upstream components of this network remain functional within these in vitro models. To support this, we transiently transfected wildtype AKT, a phospho-mimetic AKT (AKTSer473D), wildtype FOXO3a or a phosphor-mutant FOXO3a (FOXO3a-AAA) into our isogenic cell lines ( Supplementary Fig. 3a,b ). We note that the over-expression of either AKTSer473D or FOXO3a-AAA negated the TRIB2-dependent resistance to BEZ235 treatment. In contrast, over-expression of either WT AKT or FOXO3a did not. For this we conclude that TRIB2-mediated resistance was AKT-dependent via FOXO3a. Interestingly there was no significant difference in protein expression for PDK1, pSer241-PDK1, RAPTOR, pSer792-RAPTOR, p70S6K and only a slightly increased level of pThr389-p70S6K correlated with TRIB2 expression ( Supplementary Fig. 4 ) Taken together we conclude that TRIB2-conferred resistance to PI3K and mTORC1 inhibitors is independent of PDK1 and p70S6K. 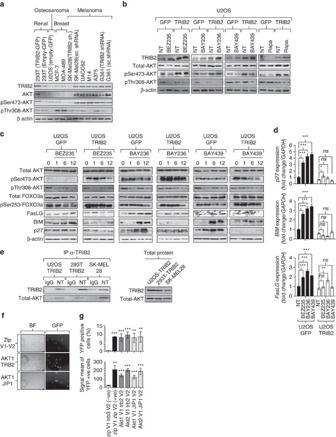Figure 2: TRIB2 protein expression correlates with AKT activation status and response to PI3K inhibition. (a) TRIB2 protein levels correlate with AKT-Ser473 phosphorylation in a broad range of modelin vitromodels. Representative images showing 100 μg (TRIB2), 50 μg (AKT-Ser473) total protein loaded per lane separated by 10% SDS–PAGE. sc indicates scramble shRNA within the indicated cell lines. (b) Immunoblot profiles for matched isogenic TRIB2 cell lines for the AKT signalling network. High-TRIB2 expression correlated with significantly increased post-translational modification(s) of downstream AKT targets. (c) Temporal inhibition of PI3K-dependent signalling following exposure to PI3K inhibitors. Total protein lysate of 50–200 μg was loaded per lane and separated by 6–12% SDS–PAGE. (d) FOXO3a-dependent gene expression was evaluated following 12 h treatment with PI3K inhibitors. NT indicates no treatment. *P<0.05 **P<0.01, ***P<0.005 by two-way ANOVA. Data represent the±s.d.nsindicates that the comparison was not statistically significant. (e) (left) Co-immunoprecipitation of TRIB2 or total AKT1 from indicated cell lines, (500 μg total protein lysate immunoprecipitated per lane) and separated by 8–12% SDS–PAGE. (right) Total protein levels in each indicated cell line for co-IP targets (100 μg total protein loaded per lane and separated by 8–12% SDS–PAGE). (f) Representative yellow fluorescent protein (YFP) complementation microscopy analysis assay for the assessment of the interaction between AKT1/2 and TRIB2. The leucine zipper Venus1 and Venus2 (ZIPV1-V2) constructs were used as a positive control, while the combination of TRIB3 V2 and V1 are our negative control. AKT1/2 JIP1 constructs were an additional control of a known AKT protein/protein complex. BF indicates bright field. (g) (top) Percentage of YFP positive cells determined by FACS. (bottom) Mean fluorescent intensity of YFP positive cells. One-way ANOVA with Dunnett’s multiple comparison test,n=4 (*P≤0.05, **P≤0.01, ***P≤0.001). All analysis was conducted compared to zipV1trib3V2 (lane 1). Figure 2: TRIB2 protein expression correlates with AKT activation status and response to PI3K inhibition. ( a ) TRIB2 protein levels correlate with AKT-Ser473 phosphorylation in a broad range of model in vitro models. Representative images showing 100 μg (TRIB2), 50 μg (AKT-Ser473) total protein loaded per lane separated by 10% SDS–PAGE. sc indicates scramble shRNA within the indicated cell lines. ( b ) Immunoblot profiles for matched isogenic TRIB2 cell lines for the AKT signalling network. High-TRIB2 expression correlated with significantly increased post-translational modification(s) of downstream AKT targets. ( c ) Temporal inhibition of PI3K-dependent signalling following exposure to PI3K inhibitors. Total protein lysate of 50–200 μg was loaded per lane and separated by 6–12% SDS–PAGE. ( d ) FOXO3a-dependent gene expression was evaluated following 12 h treatment with PI3K inhibitors. NT indicates no treatment. * P <0.05 ** P <0.01, *** P <0.005 by two-way ANOVA. Data represent the±s.d. ns indicates that the comparison was not statistically significant. ( e ) (left) Co-immunoprecipitation of TRIB2 or total AKT1 from indicated cell lines, (500 μg total protein lysate immunoprecipitated per lane) and separated by 8–12% SDS–PAGE. (right) Total protein levels in each indicated cell line for co-IP targets (100 μg total protein loaded per lane and separated by 8–12% SDS–PAGE). ( f ) Representative yellow fluorescent protein (YFP) complementation microscopy analysis assay for the assessment of the interaction between AKT1/2 and TRIB2. The leucine zipper Venus1 and Venus2 (ZIPV1-V2) constructs were used as a positive control, while the combination of TRIB3 V2 and V1 are our negative control. AKT1/2 JIP1 constructs were an additional control of a known AKT protein/protein complex. BF indicates bright field. ( g ) (top) Percentage of YFP positive cells determined by FACS. (bottom) Mean fluorescent intensity of YFP positive cells. One-way ANOVA with Dunnett’s multiple comparison test, n =4 (* P ≤0.05, ** P ≤0.01, *** P ≤0.001). All analysis was conducted compared to zipV1trib3V2 (lane 1). Full size image TRIB2 and AKT interact and form a protein-protein complex FOXOs have been shown to be the major transcriptional effectors following PI3K inhibition [13] and consistent with this finding, we observe significantly elevated pSer235-FOXO3a protein levels and a concomitant suppression of FOXO-dependent gene expression in cells with high-TRIB2 protein expression ( Fig. 2c,d ). Our data raise the hypothesis that TRIB2-dependent FOXO suppression is indirect and rather, could be mediated via p473-AKT1 activation. To address this hypothesis we investigated the mTORC2/AKT/FOXO3a cascade as mTORC2 is responsible for the phosphorylation of ser473 within AKT1 (ref. 14 ). We questioned if there was physical interaction between TRIB2, AKT1 and pThr1135-RICTOR using co-immunoprecipitation and protein fragment complementation assays [15] , [16] , [17] . The results showed a strong interaction between TRIB2 and AKT1 but could not observe TRIB2/RICTOR binding ( Fig. 2e,f ). Strikingly, the TRIB2/AKT1 complex (including the intensity of the interaction) was as strong as the known AKT1/JIP1 interaction [18] . Developing these findings further, we addressed the functional importance of FOXO and RICTOR in TRIB2-dependent drug resistance. Four different shRNA constructs were used to stably silence FOXO3a expression ( Supplementary Fig. 5 ). The depletion of FOXO3a expression significantly increased in vitro resistance to PI3K inhibitors regardless of TRIB2 status ( Fig. 3a ). Furthermore, FOXO3a depletion abolished the TRIB2-dependent difference, we previously observed for FOXO-regulated gene transcription in our isogenic cell lines ( Fig. 3b ). In addition to phosphorylating and directing FOXO3a for proteasome mediated degradation, AKT1 can also suppress apoptosis by activating the E3 ubiquitin ligase mouse double minute 2 homologue (MDM2), thus inhibiting p53-mediated apoptosis [6] , [19] . To analyse the role of TRIB2 within this ‘arm’ of the AKT network, we broadened our study to include first line chemotherapeutics known to act through p53 that are independent of FOXO ( Fig. 3c , Supplementary Fig. 6 ). Remarkably, TRIB2 over expression significantly increased cell resistance to dacarbazine (DTIC), gemcitabine and 5-fluorouracil (5-FU) induced cell death independent of FOXO. Accordingly, high-TRIB2 expression was associated with notably elevated pSer166-MDM2 protein levels ( Fig. 3d ). Therefore, we questioned whether p53 regulation was disrupted by increased TRIB2 protein levels. We found that high-TRIB2 protein expression correlated with a significantly lower p53 protein level in the absence of DNA damage or cellular stress consistent with increased MDM2 activity ( Fig. 3d ). Concomitant to this reduced p53 protein level, we observed the diminished expression of p53 target genes including p21, MDM2, Bax and PUMA ( Fig. 3e ). Altogether these data highlight the involvement of TRIB2 within the PI3K signalling network, affecting cell line resistance to various anti-cancer agents by activating AKT1, inhibiting FOXO and p53. 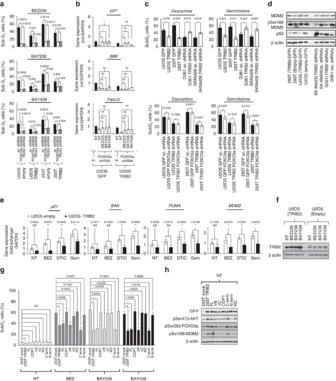Figure 3: TRIB2-mediated resistance to chemotherapeutics is via AKT activation, suppressing FOXO3a and p53. (a) Matched isogenic TRIB2 cell line FACS analysis following the knockdown of FOXO3a and subsequent exposure to BEZ235, BAY236 (copanlisib) or BAY439 (BAY1082439) (n=6).Pvalues are indicated for each comparison by two-way ANOVA and data represent the mean±s.d. (b) Quantitative real time PCR (qRT-PCR) analysis of FOXO3a-dependent gene expression after FOXO3a knockdown and isogenic cell line treatment for 24 h with PI3K inhibitors (n=6), (*P≤0.05, **P≤0.01 and were analysed by two-way ANOVA). Data represent the mean±s.d. (c) Matched isogenic TRIB2 cell line FACS analysis after 72 h exposure to various chemotherapeutics (n=6).Pvalues are indicated for each comparison and data represent the mean±s.d. (d) I Representative immunoblot analysis showing 50 μg (MDM2), 100 μg (MDM2-Ser166), 50 μg (p53) total protein lysate per lane separated by 6–10% SDS–PAGE. (e) p53-dependent gene expression was evaluated following TRIB2 isogenic cell line treatment with each indicated chemotherapeutic agent for 24 h.Pvalues are shown for comparison by 2-way ANOVA (*P≤0.05, **P≤0.001, ***P≤0.0001) and data shown indicates mean±s.d. (f) Representative immunoblot analysis showing TRIB2 protein expression (100 μg total protein loaded per lane) following exposure to each indicated PI3K inhibitor. (g) FACS analysis of 293T cells after transfection of each TRIB2 construct and subsequent exposure to BEZ235, BAY236 (BAY 80-6946) or BAY439 (BAY1082439) (n=6) for 72 h.Pvalues are indicated for each comparison by two-way ANOVA and data represent the mean±s.d.Pvalues are shown for each comparison where no significant difference was noted. Data was analysed by 2-way ANOVA *P≤0.05, **P≤0.001. (h) Representative immunoblot analysis showing 50 μg (GFP), 100 μg (AKT-Ser473), 100 μg (FOXO3a-Ser253), 100 μg (MDM2-Ser166) protein expression 48 h post-transfection of the indicated GFP tagged TRIB2 plasmid constructs. Figure 3: TRIB2-mediated resistance to chemotherapeutics is via AKT activation, suppressing FOXO3a and p53. ( a ) Matched isogenic TRIB2 cell line FACS analysis following the knockdown of FOXO3a and subsequent exposure to BEZ235, BAY236 (copanlisib) or BAY439 (BAY1082439) ( n =6). P values are indicated for each comparison by two-way ANOVA and data represent the mean±s.d. ( b ) Quantitative real time PCR (qRT-PCR) analysis of FOXO3a-dependent gene expression after FOXO3a knockdown and isogenic cell line treatment for 24 h with PI3K inhibitors ( n =6), (* P ≤0.05, ** P ≤0.01 and were analysed by two-way ANOVA). Data represent the mean±s.d. ( c ) Matched isogenic TRIB2 cell line FACS analysis after 72 h exposure to various chemotherapeutics ( n =6). P values are indicated for each comparison and data represent the mean±s.d. ( d ) I Representative immunoblot analysis showing 50 μg (MDM2), 100 μg (MDM2-Ser166), 50 μg (p53) total protein lysate per lane separated by 6–10% SDS–PAGE. ( e ) p53-dependent gene expression was evaluated following TRIB2 isogenic cell line treatment with each indicated chemotherapeutic agent for 24 h. P values are shown for comparison by 2-way ANOVA (* P ≤0.05, ** P ≤0.001, *** P ≤0.0001) and data shown indicates mean±s.d. ( f ) Representative immunoblot analysis showing TRIB2 protein expression (100 μg total protein loaded per lane) following exposure to each indicated PI3K inhibitor. ( g ) FACS analysis of 293T cells after transfection of each TRIB2 construct and subsequent exposure to BEZ235, BAY236 (BAY 80-6946) or BAY439 (BAY1082439) ( n =6) for 72 h. P values are indicated for each comparison by two-way ANOVA and data represent the mean±s.d. P values are shown for each comparison where no significant difference was noted. Data was analysed by 2-way ANOVA * P ≤0.05, ** P ≤0.001. ( h ) Representative immunoblot analysis showing 50 μg (GFP), 100 μg (AKT-Ser473), 100 μg (FOXO3a-Ser253), 100 μg (MDM2-Ser166) protein expression 48 h post-transfection of the indicated GFP tagged TRIB2 plasmid constructs. Full size image It has been previously reported that TRIB2 associated with and inhibited the transcription factor CCAAT/enhancer-binding protein alpha (C/EBPα) [11] . Gene expression analysis in our isogenic cell lines revealed that high-TRIB2 expression leads to reduced number of C/EBPα transcripts and the downregulation of C/EBPα target genes ( Supplementary Table 5 ), which might contribute to the response to drug treatment. The COP1 domain of TRIB2 is required for AKT activation To identify directly the TRIB2 functional domains that effect AKT activation, FOXO3a suppression and confer resistance to PI3K inhibitors, we employed a variety of mutated TRIB2 proteins ( Supplementary Fig. 7a ) [20] . The ΔC, kinase domain (KD), ΔCOP1 and the N-terminal TRIB2 constructs did not confer resistance to any of the PI3K inhibitors tested ( Fig. 3g ). However, the full length, ΔN and the C-terminal constructs did confer resistance to each of the investigated therapeutics indicating that the COP1 region could be driving cell line resistance. In ΔC, KD, ΔCOP1 and N-terminal transfected cells, we observe little to no change in the level of pSer473-AKT1. In contrast, in untreated cells transfected with full length, ΔN or the C-terminal TRIB2 constructs, the levels of pSer473-AKT1, pSer253-FOXO3a and pSer166-MDM2 increased significantly ( Fig. 3h ). Alongside, these phosphorylation events we observed a significant reduction of FOXO3a-dependent gene and protein expression ( Supplementary Fig. 7b,c ). Taken together, these data support that the TRIB2 COP1 domain promotes AKT activation repressing FOXO3a and p53 activity, thereby fuelling cellular resistance to PI3K inhibitor regimes. TRIB2 protein confers in vivo resistance to BEZ235 treatment To address if TRIB2 over expression ablated tumour regression following the in vivo administration of PI3K inhibitors, we established isogenic 293T subcutaneous tumours in the flanks of NOD/Scid mice. Tumours formed equivalently in these mice irrespective of TRIB2 status. The daily oral administration of BEZ235 resulted in the regression of 293T-GFP xenograft tumours and a statistically significant increase in survival. In contrast, 293T-TRIB2 tumours were highly resistant to treatment, correlating with our i n vitro studies indicating that TRIB2 over expression significantly reduced the effectiveness of BEZ235 treatment in vivo ( Fig. 4a,b ). To further support our in vitro analysis, we also collected (where possible) tumours from each mouse and evaluated the protein expression profiles ( Fig. 4c ). We note that while there was variable overall protein expression within the various treatment groups, that 293T-TRIB2 BEZ235 treated tumours had significantly higher total and pSer473 AKT compared to 293T-GFP BEZ235 treated tumours. In contrast 293T-TRIB2 BEZ235 treated tumours show attenuated FasLG protein expression. 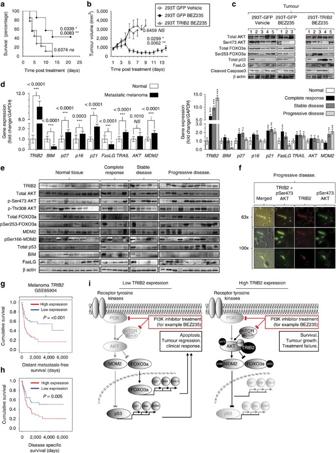Figure 4: TRIB2-conferred resistance to PI3K inhibitorsin vivoandex vivo andcorrelates with poor clinical prognosis. (a) Kaplan–Meier analysis of isogenic TRIB2 cell lines grow subcutaneously inNOD/Scidmice treated with vehicle (n=7), of BEZ235 (n=7). The presence of TRIB2 significantly reduced survival (log rankP=0.033) when treated daily with BEZ235. (b) TRIB2 overexpressing 293T tumours (n=7) show little to no response to daily administration of BEZ235 compared to isogenic lines with endogenous (low,n=7) TRIB2 expression. (c) Representative immunoblot analysis of key proteins of interest fromin vivotreated tumours. Only three tumours were present from the 293T-empty-BEZ235 treatment group. Red line (on 293-TRIB2 treated immunoblots highlight bands from the same membrane that were spliced due to lane gaps left on the original full immunoblot. Original full membranes are provided inSupplementary Information;Supplementary Fig. 19). (d) (left panel) Quantitative real time PCR (qRT-PCR) analysis of gene expression inex vivometastatic melanoma samples (n=20) versus normal control tissue (n=10). Data were analysed by two-way ANOVA) and values represent the mean±s.d. (right panel), Quantitative real time PCR (qRT-PCR) analysis of gene expression inex vivometastatic melanoma samples (n=20) versus normal control tissue (n=10) classified by clinical response to first line chemotherapy (complete responsen=5, stable diseasen=5 or progressive diseasen=10). Data were analysed by two-way ANOVA) *P≤0.05, **P≤0.01, ***P≤0.001) and values represent the mean±s.d. (e) Representative immunoblot analysis of the AKT signalling cascade fromex vivometastatic melanoma samples compared to normal tissue samples. (f) Representative immunofluorecent images of metastatic melanoma dual stained for TRIB2 and pSer473-AKT1 demonstrating co-staining and interaction. (g) Kaplan–Meier analysis from melanoma patients in the GSE65904 dataset classified based on low (≥1.5 fold) or high (≥2.5 fold)TRIB2expression. Log-rank tests reveal thatTRIB2expression is highly significant for patient prognosis with median survival for low (4,450 days) and high (394 days) expression respectively. (h) Kaplan–Meier analysis for metastasis-free survival based on low (≥1.5 fold) or high (≥2.5 fold)TRIB2expression (i) Proposed model of TRIB2-mediated drug resistance. Figure 4: TRIB2-conferred resistance to PI3K inhibitors in vivo and ex vivo and correlates with poor clinical prognosis. ( a ) Kaplan–Meier analysis of isogenic TRIB2 cell lines grow subcutaneously in NOD/Scid mice treated with vehicle ( n =7), of BEZ235 ( n =7). The presence of TRIB2 significantly reduced survival (log rank P =0.033) when treated daily with BEZ235. ( b ) TRIB2 overexpressing 293T tumours ( n =7) show little to no response to daily administration of BEZ235 compared to isogenic lines with endogenous (low, n =7) TRIB2 expression. ( c ) Representative immunoblot analysis of key proteins of interest from in vivo treated tumours. Only three tumours were present from the 293T-empty-BEZ235 treatment group. Red line (on 293-TRIB2 treated immunoblots highlight bands from the same membrane that were spliced due to lane gaps left on the original full immunoblot. Original full membranes are provided in Supplementary Information ; Supplementary Fig. 19 ). ( d ) (left panel) Quantitative real time PCR (qRT-PCR) analysis of gene expression in ex vivo metastatic melanoma samples ( n =20) versus normal control tissue ( n =10). Data were analysed by two-way ANOVA) and values represent the mean±s.d. (right panel), Quantitative real time PCR (qRT-PCR) analysis of gene expression in ex vivo metastatic melanoma samples ( n =20) versus normal control tissue ( n =10) classified by clinical response to first line chemotherapy (complete response n =5, stable disease n =5 or progressive disease n =10). Data were analysed by two-way ANOVA) * P ≤0.05, ** P ≤0.01, *** P ≤0.001) and values represent the mean±s.d. ( e ) Representative immunoblot analysis of the AKT signalling cascade from ex vivo metastatic melanoma samples compared to normal tissue samples. ( f ) Representative immunofluorecent images of metastatic melanoma dual stained for TRIB2 and pSer473-AKT1 demonstrating co-staining and interaction. ( g ) Kaplan–Meier analysis from melanoma patients in the GSE65904 dataset classified based on low (≥1.5 fold) or high (≥2.5 fold) TRIB2 expression. Log-rank tests reveal that TRIB2 expression is highly significant for patient prognosis with median survival for low (4,450 days) and high (394 days) expression respectively. ( h ) Kaplan–Meier analysis for metastasis-free survival based on low (≥1.5 fold) or high (≥2.5 fold) TRIB2 expression ( i ) Proposed model of TRIB2-mediated drug resistance. Full size image TRIB2 status corresponds to clinical outcome We next questioned if these findings are representative of the clinical situation. We collected tumour tissue samples from patients with melanoma, pancreatic and colon cancer prior to standard anti-cancer therapies (DTIC, gemcitabine or paclitaxel). Compared to normal tissue samples, TRIB2 transcription and TRIB2 protein expression was significantly increased in metastatic melanoma, primary colon and primary pancreatic cancer tissue samples ( Fig. 4d–f ; Supplementary Fig. 8 ). We did not detect a significant increase in either TRIB1 or TRIB3 expression in any of the samples analysed ( Supplementary Fig. 9 ). Concomitant with TRIB2 status, we found that pSer473-AKT1 and pSer253-FOXO3a protein levels were significantly higher, while the transcript and protein levels of the FOXO-dependent genes BIM , FasLG and TRAIL were significantly lower in ex vivo melanoma samples compared to normal control tissue samples. Importantly, when we classified our samples based on the clinical outcome of the respective patients, we noted that TRIB2 expression correlated with a significantly worse prognosis ( Fig. 4d ). We next investigated whether our transcription data correlated with protein levels. First, TRIB2 protein expression was distinctly increased in melanoma tissue samples compared to normal skin and second, the highest TRIB2 protein expression was observed in melanoma tissues samples from patients with a poor clinical outcome ( Fig. 4e ; Supplementary Fig. 10 ). We next questioned whether there was also a de-regulated AKT signalling within our clinical samples. Consistent with both our in vitro and in vivo data, we observed significantly elevated total AKT, pSer473-AKT1, pSer253-FOXO3a and pSer166-MDM2 and no significant difference regarding pThr308-AKT1. Our study also demonstrated that pSer473-AKT1 and pSer253-FOXO3a levels correlated with melanoma patient prognosis. Further examination of AKT in our clinical samples revealed that TRIB2 and pSer473-AKT1 co-localize in melanoma cells from patients with progressive disease ( Fig. 4f ). Finally, we examined the clinical significance of our ex vivo data within large patient cohorts. Melanoma, colon and pancreatic tumour tissue samples were analysed based on TRIB2 expression (low ≥1.5, high ≥2.5 versus normal tissue expression) and Kaplan–Meier survival curves plotted. For melanoma and colon cancer patients, high- TRIB2 expression correlated with a significantly worse clinical outcome ( Fig. 4g,h ; Supplementary Fig. 11 ). For pancreatic cancer, there was only a strong trend for high- TRIB2 expression, primarily due to the extremely poor overall prognosis exhibited in pancreatic cancer patients. We further analysed the GSE65904 data set [21] addressing several clinical parameters, which when combined with TRIB2 expression were used to determine if TRIB2 expression was dependent or independent of these prognostic parameters. Using a multivariate cox regression model we note that TRIB2 transcription is a prognostic factor, independent of disease stage, tissue involvement, age and gender ( Supplementary Tables 6 and 7 ). Furthermore, survival data from the GSE65904 dataset revealed a highly significant TRIB2 -dependent distant metastasis-free survival time or disease-specific survival time response ( Fig. 4g,h ). Interestingly, this correlation to patient prognosis was only observed for TRIB2 and not for TRIB1 or TRIB3 ( Supplementary Fig. 12a–f ). Overall, our data reveal novel and important mechanisms of TRIB2-dependent intrinsic resistance to standard chemo therapies and PI3K inhibitors. A patient tumour population with a high-TRIB2 protein level prior to treatment would be predicted to respond poorly to these treatments by promoting PI3K/PDK1-independent AKT activation ( Fig. 4i ). This AKT activation (and subsequent inactivation of FOXO and p53) may also be highly relevant for other therapeutics that target the upstream PI3K/AKT network such as trastuzumab approved for the treatment of breast and gastric cancers and cetuximab for the treatment of colon cancer [22] . Thus, patients whose tumours display high-TRIB2 expression may not benefit from specific PI3K inhibitor therapeutics, rendering TRIB2 as a suitable biomarker predicting treatment outcome and selecting patients for individualized therapy. Furthermore, TRIB2 inhibitors might synergize with current therapies targeting the PI3K/AKT pathway hereby improving treatment outcome and patient survival. Online Content, Any additional Methods, Extended Data display items and Source Data are available in the online version of the paper; references unique to these sections appear only in the online paper. Tissue samples Surgically excised tumour tissue samples from colon cancer primaries, pancreatic cancer primaries and melanoma metastases were obtained from patients prior to first-line systemic therapy. Core tumour samples of colon carcinoma were obtained from patients with colon cancer at the time of their surgery. For each colon cancer patient, a section of matched normal colon tissue was extracted adjacent to the tumour site. Pancreatic tumour tissue (and matched normal tissue) was obtained during surgery (employing the Whipple surgical methodology). Melanoma tumour samples were obtained from metastatic lesions from patients with advanced melanoma in AJCC stage IV. Informed consent was obtained for the use of these samples. The samples were freshly frozen and cryo-preserved until processing. Before analysis, the frozen tissue samples were split into smaller sections for RNA extraction using TRI-Reagent (Sigma). The clinical data of the corresponding patients were extracted from the patient files. Cell lines and reagents The human cell lines SK-Mel28, A375, N14, G361, UACC62, M14 (melanoma), HEK293T (renal cell carcinoma), U2OS [p53 +/+ ], Soas2 [p53 −/− ] (osteosarcoma), MCF-7 and MDA-MB231 (breast cancer) were maintained in DMEM supplemented with 10% FBS (Sigma, PT) and antibiotics (Gibco, US). Cell lines were mycoplasma tested monthly within the CBMR by PCR (LookOut Mycoplasma PCR Detection Kit, SIGMA, PT). All cell lines are indicated in Supplementary Table 1 . Antibodies shown in Supplementary Table 2 were used for our immunoblots and signal visualization was achieved using a ChemidocXRS+ system (BioRad, PT). Dacarbazine (Sigma, PT), gemcitabine hydrochloride (Eli Lilly #VL7502), AKT inhibitor VIII (Calbiochem, US), BEZ235 (Novartis, US), BAY236, (BAY 80-6946) BAY439 (BAY1082439), BAY1001931 (a gift from Bayer AG, Germany), rapamycin (SIGMA, PT), actinomycin D (Sigma, PT), and cyclohexamide (Sigma, PT) and MG132 (Sigma, PT) were used at concentrations described in the text. Constructs and shRNA A 3062, bp fragment encoding the entire human Trib2 (hTRIB2) cDNA was sub-cloned into pEGFP-N1 or pIREPuro2 plasmids, (one co-expressing GFP, the other containing a V5 tag.). Full length human TRIB2 (hTRIB2, 1-343 aa), dN (63-343aa hTRIB2, dC (1-304 aa) hTRIB2, KD (63-304 aa) hTRIB2, NT (ΔCT, 1–250 aa) hTRIB2, CT (ΔNT, 270-343 aa) hTRIB2 and ΔCOP1 hTRIB2 were kindly provided by W.S. Pear. Each was cloned into pMigR1-myc plasmid as described in ref. 20 . Full length pAKT1-S473D and pCMV6HA-mAKT1 were kindly provided by A. Newton. pECE-Foxo3a-(A)3 and pCLne-wt-Foxo3a were kindly provided by M. Greenberg. All complementary DNAs (cDNAs) were sequenced in their entirety to verify there were no mutations in any of our constructs. FOXO3a shRNA constructs originated from the NKI library, FOXO3a-826, FOXO3a-827 and FOXO3a-828 were cloned into pRetroSuper. hTRIB2 shRNA-917 or hTRIB2-918 were sub-cloned into pRetroSuper. Each construct was transfected into indicated cell lines for selection and screening. Full sequences are provided in our Supplementary Information . For our protein fragment complementation assays, cells were co-transfected with the Venus plasmid constructs [23] for AKT1 (1032-2471aa), AKT2 (1032-2477aa) or TRIB2 (1012-2042aa). YFP signal was quantified using flow cytometry (FacsCalibur, Becton Dickinson). The images of the interactions were captured by a Leica DMI 4000B inverted fluorescence microscope. Western blot analysis For the preparation of whole cell lysate, cells were harvested and lysed using RIPA buffer (50 mM Tris–HCl pH 7.4, 1% NP-40, 0.5% Na-deoxychlorate, 150 mM NaCl, 1 mM EDTA, 2 mM NaF, 2 mM NaVO 4 and 1 × protease inhibitor cocktail (PIC) (Sigma). For SDS–polyacrylamide gel electrophoresis (SDS–PAGE), protein samples were boiled for 5–10 min in protein sample buffer (50 mM Tris pH 6.8, 1% SDS, 10% glycerol, 0.01% Bromophenol Blue, β mercaptoethanol (50 μl per 950 μl sample buffer)). Following electrophoresis, proteins were transferred onto nitrocellulose membrane (BioRad). The membrane was blocked for 1 h at room temperature or overnight at 4 °C 5% BSA 0.1% tween20 blocking buffer. Primary antibodies were added to the membrane ( Supplementary Table 2 ) overnight at 4 °C or for 2 h at room temperature. Secondary antibody was added (Santa Cruz Biotechnology) at typically 1:5,000 dilution for 1 h at room temperature. Visualization of signal was achieved using a ChemiDocXRS+ Imaging System (BioRad). Full original membranes are shown in Supplementary Figs 13–25 . Co-immunoprecipitation Co-immunoprecipitations (Co-IP) were performed as described in (ref. 18 ). Cells were lysed in cold lysis buffer (50 mM Tris-Cl at pH 7.4, 150 mM NaCl, 1 mM EDTA, 1% NP-40, 0.25% sodium deoxycholate, protease inhibitor mixture). Cell extracts (500 μg) were incubated with the first antibodies ( Supplementary Table 2 ) or control normal IgG on a rotator overnight at 4 °C, followed by addition of protein G magnetic beads (Invitrogen) for 2 h at 4 °C. Beads were then washed four times using the lysis buffer. The immune complexes were subjected to SDS–PAGE followed by immunoblotting with the secondary antibody. Quantitative Real time PCR (qRT-PCR) Total RNA was extracted by using TRI-reagent (Sigma, PT). cDNA was generated using NZY First-Strand cDNA Synthesis Kit (NZYTech, PT). Real Time PCR was performed on a BioRad CFX96 quantitative real time PCR machine using the SYBR Green JumpStart master mix (Sigma, PT). The primer sequences (NZYTech, PT) for measuring p16, p27, FasLG, Bim, TRAIL, p21, Bax, PUMA, MDM2, TRIB1, TRIB2, TRIB3 and GAPDH are shown in Supplementary Table 3 . Data analysis was carried out using the 2 −ΔΔCT method [24] . Flow cytometric cell cycle analysis Cells were grown to 70% confluence. Cells were mock treated/exposed to each compound for the time points indicated. Samples were collected, washed (PBS) and fixed (70% ethanol). Ethanol was removed and samples were resuspended in PBS. Propidium iodide (2.5 mg ml) was added to each sample. Samples were run on a Fluorescence Activated Cell Scanner (FACS) and the percentage populations (sub-G 1 , G 1 , S and G 2 phases) determined. 50,000 total events were scored per study Data was analysed using Infinicyt (Cytognos). In vivo studies In vivo efficacy studies were performed using 293T-GFP and 293T-TRIB2 cells injected subcutaneously in the flank of female NOD/SCID mice. Animals were treated with either vehicle alone (20% N-Methyl-2-pyrrolidone (NMP) 80% polyethylene glycol (PEG) 300) or BEZ235 (30 mg kg −1 by oral gavage. Treatment was administered daily for the indicated length of time. Tumours were measured manually by calliper daily. All in vivo modelling was carried out according to guidelines, regulations set out in Portuguese law (Portaria 1005/02 and Portaria 1131/97), which transcribes the European Guideline 86/609/EC and approved by the CBMR Biotério ethics board. Fixing and staining samples for immunofluorescence To fix samples/cells, slides/coverslips were fixed and permeabilised for 15 min in dry methanol at −20 °C and rehydrated in PBS. Samples/cells were blocked (donkey serum 1:30) for 1 h at 37 °C in a humified chamber incubated with primary antibody (either Anti-pSer473AKT1 or TRIB2) for 1 h at 37 °C in a humified chamber followed by PBS washing and incubation with a fluorescent secondary antibody (Molecular Probes A21207 or A11055) for 1 h at 37 °C in a humified chamber. Antibody solutions were made in PBS (Sigma). Following labelling procedures, samples/cells were mounted on glass slides in Clear Mount mounting solution (Invitrogen). Statistical analysis Statistical significance was assessed by two-way analysis of variance (ANOVA) or the two-tailed Students t -test. Statistical significance was defined as P ≥0.05. Results are expressed as the mean±s.d. or s. e. of the mean (s.e.m.) and are described in each figure legend when applied. Data availability The authors declare that the data supporting the findings of this study are available within the paper and its Supplementary Information files. How to cite this article: Hill, R. et al . TRIB2 confers resistance to anti-cancer therapy by activating the serine/threonine protein kinase AKT. Nat. Commun. 8, 14687 doi: 10.1038/ncomms14687 (2017). Publisher's note : Springer Nature remains neutral with regard to jurisdictional claims in published maps and institutional affiliations.